Regulating proton-coupled electron transfer for efficient water splitting by manganese oxides at neutral pH Manganese oxides have been extensively investigated as model systems for the oxygen-evolving complex of photosystem II. However, most bioinspired catalysts are inefficient at neutral pH and functional similarity to the oxygen-evolving complex has been rarely achieved with manganese. Here we report the regulation of proton-coupled electron transfer involved in water oxidation by manganese oxides. Pyridine and its derivatives, which have p K a values intermediate to the water ligand bound to manganese(II) and manganese(III), are used as proton-coupled electron transfer induction reagents. The induction of concerted proton-coupled electron transfer is demonstrated by the detection of deuterium kinetic isotope effects and compliance of the reactions with the libido rule. Although proton-coupled electron transfer regulation is essential for the facial redox change of manganese in photosystem II, most manganese oxides impair these regulatory mechanisms. Thus, the present findings may provide a new design rationale for functional analogues of the oxygen-evolving complex for efficient water splitting at neutral pH. The development of efficient catalysts for the oxidation of water to molecular oxygen has long been the focus of intense research [1] , [2] , [3] , [4] , [5] , [6] , [7] , [8] , [9] , [10] , [11] , [12] . Such studies are motivated by the desire to understand the water splitting process in natural systems, such as photosystem II (PSII) of oxygenic photosynthesis, and artificial photosynthetic systems designed to produce hydrogen through proton reduction or convert carbon dioxide to fuels. In nature, water oxidation proceeds with extraordinarily high catalytic activity in PSII, in which a Ca-containing tetrameric manganese cluster (CaMn 4 O 5 ) supported by bridged oxides or hydroxides and carboxylate and histidine side chains from the protein serves as the multi-electron oxidation catalyst [13] , [14] , [15] , [16] , [17] , [18] . Notably, all species capable of O 2 evolution possess a qualitatively identical reaction centres, and no metal element other than Mn has been identified in the catalytic cluster of PSII. Therefore, extensive research efforts have been aimed at developing water-oxidation catalysts composed of the abundant element Mn [19] , [20] , [21] , [22] , [23] , [24] , [25] , [26] , [27] , [28] , [29] . However, a remarkable contradiction still exists on the catalytic performance between naturally occurring and synthetic Mn catalysts, particularly under neutral pH conditions. Although bioinspired water-oxidation catalysts, particularly Mn oxides, function as effective electrocatalysts under alkaline conditions [30] , [31] , [32] , the activity of most Mn oxides is markedly reduced at neutral pH, resulting in a large electrochemical overpotential ( η ) ranging from 500 to 700 mV [32] , [33] , [34] , [35] . This high η contrasts that of the PSII tetrameric Mn cluster, which catalyzes water oxidation with an η of only 160 mV [15] , [16] , [17] . Recently, we have shown the primary origin for these sharp declines of catalytic potential of MnO 2 under neutral conditions [35] , [36] . Measurements of in-situ water-oxidation current and optical absorption have shown that electron injection from H 2 O to anodically poised MnO 2 forms Mn 3+ , which acts as a precursor for the O 2 -evolution reaction [35] , [36] . Our studies have also demonstrated that Mn 3+ disproportionates to form Mn 2+ and Mn 4+ at pH<9, and subsequent regeneration via the electrooxidation of Mn 2+ acts as the rate-determining step in the overall four-electron/four-proton reaction [35] , [36] . It is notable that the redox change of Mn from 2+ to 3+ on the surface of MnO 2 is ~1.4 V at pH<9, which forces the onset potential for water-oxidation current ( U on, j ) to remain constant at ~1.5 V irrespective of the pH. The involvement of the pH-independent step in the redox change of Mn increases η at intermediate pH, as shown in Fig. 1a , and is the primary origin for the sharp decline of catalytic potential of MnO 2 under neutral conditions. This property prohibits the successful application of Mn oxides as components of artificial photosynthetic systems. 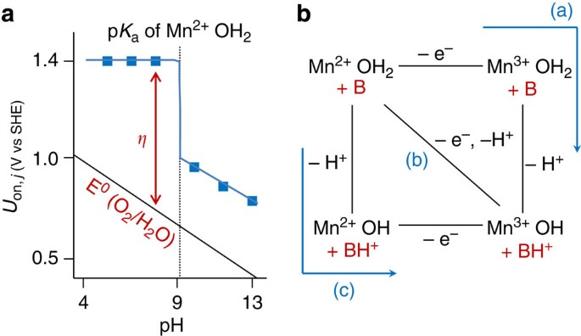Figure 1:pH-dependent water-oxidation mechanisms by MnO2electrodes. (a) Schematic illustration of the pH dependence of the onset potential (Uon,j) for water oxidation35. Under neutral conditions,Uon,jdoes not show pH dependence, whereas it exhibits a linear pH dependence at pHs above 9. The transition point from pH-independent to pH-dependent at pH~9 corresponds to the pKaof Mn2+OH2. (b) Thermodynamic cycle for the electrooxidation of Mn2+to Mn3+on the surface of MnO2electrodes. The pKavalues of the water ligand bound to Mn2+and Mn3+are 10.6 and 0.7, respectively. Thus, Mn2+and Mn3+exist as protonated and deprotonated forms, respectively, at intermediate pH. B and BH+represent the deprotonated and protonated forms, respectively, of a proton acceptor. Figure 1: pH-dependent water-oxidation mechanisms by MnO 2 electrodes. ( a ) Schematic illustration of the pH dependence of the onset potential ( U on ,j ) for water oxidation [35] . Under neutral conditions, U on ,j does not show pH dependence, whereas it exhibits a linear pH dependence at pHs above 9. The transition point from pH-independent to pH-dependent at pH~9 corresponds to the p K a of Mn 2+ OH 2 . ( b ) Thermodynamic cycle for the electrooxidation of Mn 2+ to Mn 3+ on the surface of MnO 2 electrodes. The p K a values of the water ligand bound to Mn 2+ and Mn 3+ are 10.6 and 0.7, respectively. Thus, Mn 2+ and Mn 3+ exist as protonated and deprotonated forms, respectively, at intermediate pH. B and BH + represent the deprotonated and protonated forms, respectively, of a proton acceptor. Full size image The new model explained above has suggested that the efficiency of Mn oxides as O 2 -evolution catalysts may be enhanced by regulating proton-coupled electron transfer (PCET) in the electrooxidation step of Mn 2+ to Mn 3+ . PCET is a key part of the efficient energy conversion by PSII [37] , [38] , [39] , [40] . In particular, the concerted proton-electron transfer (CPET) pathway, which involves the transfer of protons and electrons in a single concerted step, avoids charge build-up and thereby enables the redox change of the tetrameric Mn cluster in PSII over a narrow potential range (~250 mV) (refs 13 , 14 , 15 ). Therefore, it can be deduced that synthetic Mn oxides inefficiently catalyze water oxidation at neutral pH because they lack the inherent ability to manage both protons and electrons. Herein, we attempt to induce CPET on the surface of a Mn-oxide electrocatalyst and demonstrate that this rationale-based strategy improves the O 2 -evolution activity of synthetic Mn oxide in neutral medium. CPET induction by the addition of pyridine One possible way to induce CPET is the introduction of a protonation site, which has a p K a value that is intermediate between the p K a of Mn 3+ -OH 2 (0.7) and Mn 2+ -OH 2 (10.6) [41] , as predicted by the libido rule of general acid-base catalysis [42] , [43] , [44] , in close proximity to the water oxidation active site. In the course of oxidation from Mn 2+ to Mn 3+ , the p K a of the Mn center undergoes a large change that would convert an unfavourable proton-transfer reaction to a favourable one with respect to the base [40] , [41] , [42] , [43] , [44] , [45] , [46] , [47] . Therefore, the regeneration of Mn 3+ at neutral pH would be converted from a stepwise to a concerted pathway if the base accepts the proton at the PCET transition state rather than directly from Mn 2+ -OH 2 , as illustrated in Fig. 1b . In support of this speculation, recent density functional theory calculations have shown that the p K a values of terminal water ligands in biomimetic oxomanganese complexes are drastically changed upon the oxidation of Mn 2+ to Mn 3+ (refs 41 , 48 ). In addition, the agreement of the p K a value of Mn 2+ -OH 2 with the transition point between pH 9–10 for the pH-independent and -dependent activity of the electrooxidation reaction [35] ( Fig. 1a ) also provides the support for this hypothesis. Namely, at a pH greater than the p K a of Mn 2+ -OH 2 , the electrooxidation of Mn 2+ proceeds after the water ligand bound to Mn 2+ deprotonates to form Mn 2+ -OH − (path c in Fig. 1b ), whereas Mn 2+ oxidation prior to deprotonation produces the unstable intermediate Mn 3+ -OH 2 (path a in Fig. 1b ), leading to the electrooxidation of Mn 2+ -OH 2 , which is more thermodynamically unfavourable. To examine the validity of our hypothesis, the effects of pyridine on the electrocatalytic performance of Mn oxides for water oxidation and its influence on the pH dependence of U on, j were first investigated. Pyridine has a p K a (5.25) that is intermediate between that of Mn 3+ -OH 2 (0.7) and Mn 2+ -OH 2 (10.6), and exists as a deprotonated form at neutral pH. Thus, pyridine satisfies the conditions of the libido rule [42] . The current density ( j ) versus potential ( U ) curves for a synthesized MnO 2 electrocatalyst, consisting of α-MnO 2 nanoparticles deposited onto a fluorine-doped tin oxide (FTO) electrode, measured electrochemical cells operated at neutral pH with and without pyridine are shown in Fig. 2 . The amount of dissolved O 2 in the electrolyte was also monitored using a needle-type oxygen microsensor. We observed a large increase in both anodic current ( Fig. 2a ) and O 2 production ( Fig. 2b ) for the MnO 2 electrode in the presence of pyridine. The effects of pyridine were more prominent at higher concentrations, with ~200-mV negative shift in U on, j being observed at 0.5 M pyridine. Analysis of the head-space gas in the electrochemical cell containing 50 mM pyridine by gas chromatography (GC) revealed that a turnover number (evolved O 2 molecules per total Mn atoms deposited on the FTO electrode) of 17 and coulombic efficiency of 78% was reached after 90 min of electrolysis at 1.7 V, confirming that the evolved O 2 was generated from water oxidation. When electrolysis was conducted for 90 min at 1.39 V in the presence of pyridine (2.5 mM), 86 nmol of CO 2 was detected. This amount corresponds to the 4% of a coulombic efficiency if we assume the complete oxidation of pyridine to CO 2 ( Supplementary Figs 1 and 2 ). 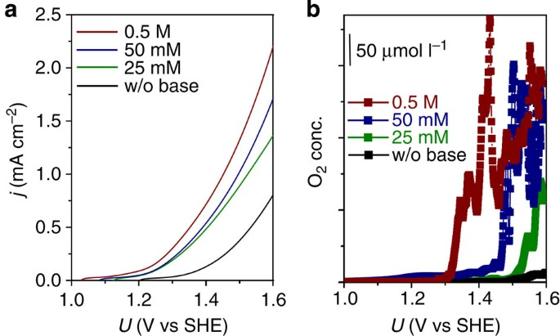Figure 2: Enhanced water oxidation by addition of pyridine. Enhanced water-oxidation activity of MnO2electrodes at pH 7.5 by the addition of pyridine. (a) Potential dependence of current density for MnO2electrodes in presence and absence of pyridine. (b) Potential dependence of dissolved O2concentration for MnO2electrodes in presence and absence of pyridine. For both (aandb) the scan rate was 10 mV s−1. Figure 2: Enhanced water oxidation by addition of pyridine. Enhanced water-oxidation activity of MnO 2 electrodes at pH 7.5 by the addition of pyridine. ( a ) Potential dependence of current density for MnO 2 electrodes in presence and absence of pyridine. ( b ) Potential dependence of dissolved O 2 concentration for MnO 2 electrodes in presence and absence of pyridine. For both ( a and b ) the scan rate was 10 mV s −1 . Full size image We next examined the pH dependence of U on, j for water-oxidation current to confirm whether CPET was induced on the surface of a Mn-oxide electrocatalyst as predicted. The electrode potential at which the current density reached 130 μA cm −2 was adopted as U on, j . In the absence of pyridine, no pH dependence of U on, j was observed at pH<10 ( Supplementary Fig. 3a ), whereas U on, j showed a clear pH dependence following the addition of pyridine into the electrochemical cell ( Supplementary Fig. 3b ). Plots of U on, j against electrolyte pH showed a pH dependence in the presence of pyridine ( Supplementary Fig. 3c,d ), demonstrating that proton transfer was involved in the rate-determining transition state for water oxidation. Notably, pyridine did not enhance water-oxidation activity at pHs higher than the p K a of Mn 2+ -OH 2 ( Supplementary Fig. 3d ), a result that is consistent with the deprotonation of the water ligand bound to Mn 2+ forming Mn 2+ -OH − at pH>10 (path c in Fig. 1b ). Similarly, when pyridine was added to the electrolyte at pH 4, almost no activity enhancement was observed, as 95% of pyridine exists as the protonated form at this pH and therefore cannot function as a proton acceptor. The results presented in Fig. 2 and Supplementary Fig. 3 are consistent with the hypothesis that pyridine accepts a proton from the water ligand bound to Mn during the PCET transition state. However, when the j − U measurements were conducted in D 2 O instead of H 2 O in the presence of 50 mM pyridine at neutral pD (pD=pH+0.4) (ref. 49 ), the kinetic isotope effect (KIE) measured at 1.37 V for j (H 2 O) and j (D 2 O) was 1.62, which is only slightly higher than the KIE obtained in the absence of pyridine (KIE=1.48). These results suggest that pyridine acts as proton acceptor in this system; however, the basicity of pyridine was not strong enough to induce the fully concerted reaction path. In other words, we consider that the electron-transfer reaction is more rapid than the transfer of the proton from the Mn-bound water ligand to pyridine and speculate that there are more suitable bases for the enhancement of catalytic activity. Regulation of PCET mechanisms by the addition of different bases In an attempt to accelerate the proton-transfer reaction, we replaced pyridine with a base that has a higher p K a value. As p K a is the index for proton-accepting ability, the addition of a base with a higher p K a was expected to promote the deprotonation of water ligand during the PCET transition state. Several pyridine derivatives, namely 3-methylpyridine (β-picoline, p K a =5.80), 4-methylpyridine (γ-picoline, 6.10), 2,6-dimethylpyridine (2,6-lutidine, 6.96), and 2,4,6-trimethylpyridine (γ-collidine, 7.48) were evaluated as candidate bases. Similar to pyridine, the p K a values of the selected derivatives are lower than that of Mn 2+ -OH 2 , meaning that the direct deprotonation of water ligands (path c in Fig. 1 ) is thermodynamically unfavourable. The j − U curves for the MnO 2 electrode in the presence of pyridine derivatives at pH 7.5 are shown in Fig. 3a . As expected, a higher catalytic activity was observed with increasing p K a of the added base. The η decreased with the increase of p K a ; for example, ~70-mV negative shift of U on, j was observed for γ-collidine relative to that for pyridine. To compensate for the concentration difference between the protonated and deprotonated forms of bases due to p K a differences, the electrolyte was prepared using a 25 mM concentration of the deprotonated base form. Therefore, the shift of U on, j that can be seen in Fig. 3a is attributable to the different proton-accepting abilities of the pyridine derivatives. GC analysis of the head-space gas revealed that the coulombic efficiency for O 2 evolution was 77% (γ-collidine), 62% (2,6-lutidine), 66% (γ-picoline) and 57% (β-picoline), and that the amount of evolved O 2 exceeded unity for all examined bases. Notably, the rate of O 2 production increased monotonically with increasing of p K a , as shown in Fig. 3b , a result that is consistent with the observed trends in the j − U curve measurements. In the case of γ-collidine, the O 2 -evolution activity of the MnO 2 electrode at pH 7.5 showed ~15fold enhancement compared with that observed in the absence of bases, reaching nearly half of the O 2 -evolution activity that was measured in alkaline medium ( Supplementary Fig. 4 ). 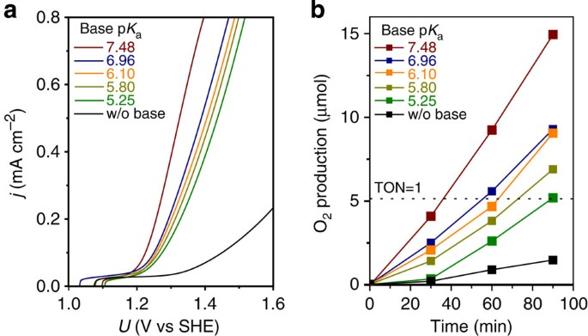Figure 3:Effects of base pKa. Effects of base pKaon electrochemical water-oxidation activity of MnO2electrodes at pH 7.5. (a) Potential dependence of current density for MnO2electrodes in the presence of pyridine (pKa=5.25; light green), β-picoline (pKa=5.80; olive green), γ-picoline (pKa=6.10; orange), 2,6-lutidine (pKa=6.96; blue) and γ-collidine (pKa=7.48; brown). A MnO2electrode without the addition of bases to the electrolyte is also depicted as a reference (black). (b) Time course of O2production observed for MnO2electrodes at an applied potential of +1.39 V versus standard hydrogen electrode (SHE) in the presence of the bases listed ina. The dashed line indicates the value corresponding to turnover number (TON)=1. The concentration of each base was adjusted to 25 mM of the deprotonated form. A MnO2electrode without the addition of bases to the electrolyte is also depicted as a reference. Figure 3: Effects of base p K a . Effects of base p K a on electrochemical water-oxidation activity of MnO 2 electrodes at pH 7.5. ( a ) Potential dependence of current density for MnO 2 electrodes in the presence of pyridine (p K a =5.25; light green), β-picoline (p K a =5.80; olive green), γ-picoline (p K a =6.10; orange), 2,6-lutidine (p K a =6.96; blue) and γ-collidine (p K a =7.48; brown). A MnO 2 electrode without the addition of bases to the electrolyte is also depicted as a reference (black). ( b ) Time course of O 2 production observed for MnO 2 electrodes at an applied potential of +1.39 V versus standard hydrogen electrode (SHE) in the presence of the bases listed in a . The dashed line indicates the value corresponding to turnover number (TON)=1. The concentration of each base was adjusted to 25 mM of the deprotonated form. A MnO 2 electrode without the addition of bases to the electrolyte is also depicted as a reference. Full size image The KIE values obtained from j − U curve measurements for the MnO 2 electrode at neutral pH (and adjusted pD=pH+0.4; ref. 49 ) were plotted as a function of base p K a ( Fig. 4a ). The concentration of the deprotonated form of bases was adjusted to 25 mM. It can be seen that the KIEs increased monotonically from 1.6 to 2.7 as the base p K a increased from 5.25 to 7.48. The KIE is a rough measure of the position of the transition state along the reaction coordinate for proton transfer [50] . Large KIEs are expected for a reaction with nearly symmetrical transition states, as the activated complex has the proton almost equally shared between the reactant and product. Meanwhile, smaller effects are observed as the transition state moves towards reactant, as very little deprotonation has occurred at transition state. Therefore, the increase of KIEs with the base p K a demonstrates that bases with a stronger proton extracting property increase the extent of deprotonation of the water ligand bound to a Mn center at the rate-determining transition state. Moreover, the pH dependence of U on, j at pH<9 became more prominent with the increasing p K a of the base ( Fig. 4b and Supplementary Fig. 5 ). For example, the shift per pH unit increased from ~25 mV for pyridine to 60 mV for γ-collidine ( Supplementary Fig. 6 ). The latter value indicates that the η for water-oxidation reaction is almost constant irrespective of a solution pH higher than p K a of γ-collidine ( Supplementary Fig. 5 ). Thus, the observed increase in KIE and the slope of pH dependence with base p K a ( Fig. 4 ), together with the concomitant enhancement of the water-oxidation activity of the MnO 2 electrode ( Fig. 3 ), demonstrate the successful induction of CPET in the electrocatalytic water oxidation by MnO 2 . 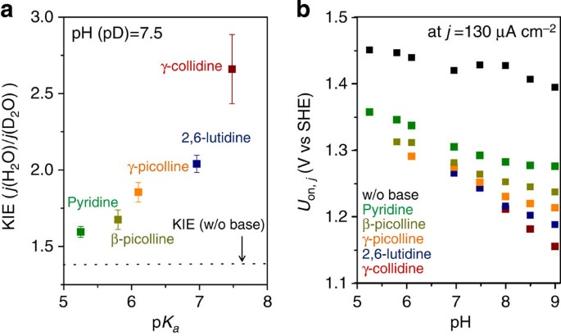Figure 4: Regulation of PCET mechanisms by the addition of bases. (a) Plot of KIE as a function of the pKaof the indicated bases at pH (pD) 7.5 at 1.29 V versus SHE. The measured pH value in D2O was converted to pD value using the equation—pD=measured pH+0.4. Base concentration: 25 mM of deprotonated form. (b) Plot of pH versus potential showing the pH dependence of the onset potential (Uon,j) defined at 130 μA cm−2for water oxidation in the presence of the indicated bases at pHs ranging from 5 to 9. Figure 4: Regulation of PCET mechanisms by the addition of bases. ( a ) Plot of KIE as a function of the p K a of the indicated bases at pH (pD) 7.5 at 1.29 V versus SHE. The measured pH value in D 2 O was converted to pD value using the equation—pD=measured pH+0.4. Base concentration: 25 mM of deprotonated form. ( b ) Plot of pH versus potential showing the pH dependence of the onset potential ( U on, j ) defined at 130 μA cm −2 for water oxidation in the presence of the indicated bases at pHs ranging from 5 to 9. Full size image We have demonstrated for the first time the regulation of PCET mechanisms involved in water oxidation by Mn oxides. Because the oxidation of Mn from 2+ to 3+ is associated with a large change in p K a , the potential of pyridine and its derivatives as a CPET-induction reagents could be evaluated based on the libido rule of general acid-base catalysis. The induction of the CPET reaction by the addition of γ-collidine was confirmed by the clear pH dependence of U on, j , which was shifted by ~60 mV, and the pronounced KIE. While the detection of KIE and compliance of the reactions with the libido rule indicated the successful regulation of PCET mechanisms, the shift of U on, j with pH in the presence of base is not explained directly by a simple model where the base is the proton acceptor. As the reaction rate of CPET is a function of the concentration of the proton acceptor, the rate is expected to be pH-independent when the concentration of deprotonated forms of base is constant. In this point of view, it is reasonably considered that the pH-dependent rate in the presence of base at the pH higher than base p K a observed in Fig. 4b could arise from the change of the rate constant for CPET. Yet it should also be noted that the base has the possibility to affect several elementary steps other than the oxidation of Mn from 2+ to 3+ in a course of electrocatalytic water oxidation. The regulation of PCET mechanisms is essential for the redox state change of the tetrameric Mn cluster in the Kok cycle of PSII and is likely promoted by amino acids whose p K a varies according to the redox state of the Mn cluster [37] , [38] , [39] . However, most bioinspired water-oxidation catalysts, particularly Mn oxides, lack such a specific regulatory mechanism, as demonstrated by the sharp decline of O 2 -evolution activity under neutral conditions for most Mn oxides reported to date [30] , [31] , [32] , [33] , [34] , [35] . Therefore, we consider that the regulation of PCET, as described in the present study, is an effective approach to lower the η for water oxidation by Mn oxides in neutral media designed for artificial photosynthesis, and will lead to new understanding for the marked difference in catalytic performance between naturally occurring and synthetic Mn catalysts at physiological pH. Synthesis procedure of α-MnO 2 α-MnO 2 powder was prepared as previously described [51] . Briefly, 1.10 g potassium permanganate (KMnO 4 ) was dissolved in 20 ml double-distilled water and the resulting mixture was stirred for 30 min at 60 °C. Separately, 1.55 g manganese (II) chloride tetrahydrate (MnCl 2 ·4 H 2 O) was added to 25 ml of a 2 M acetic acid aqueous solution, which was then stirred for 20 min at room temperature. The MnCl 2 solution was added to the KMnO 4 solution, and the resulting mixture was stirred for 2 h at 80 °C. The formed particles were collected and washed several times with doubled-distilled water. The samples were dried overnight at 60 °C and then used for preparing electrodes. All chemical reagents were obtained from Wako and utilized without further purification. Electrode preparation Particulate α-MnO 2 film electrodes were prepared using a spray deposition method, as previously described [35] . Briefly, 75 mg of the prepared MnO 2 powder sample was suspended in 20 ml water by sonication at an amplitude of 15 W for 30 min with a homogenizer (S4000, Qsonica). The suspension was diluted to 100 ml with water and was then sprayed onto a clean conducting glass substrate (FTO-coated glass, resistance: 20 Ω per square, size: 30 mm × 30 mm; SPD Laboratory, Inc.) at 200 °C using an automatic spray gun (Lumina, ST-6). After coating, the electrodes were washed thoroughly with distilled water. The amount of deposited MnO 2 was ~0.14 mg cm −2 . Electrochemical water oxidation Current density ( j ) versus potential ( U ) curves were obtained with a commercial potentiostat and potential programmer (HZ-5000, Hokuto Denko), using a Pt wire as the counter electrode and an Ag/AgCl/KCl (saturated) electrode as the reference electrode. The electrolyte solution (0.5 M Na 2 SO 4 ) was prepared using highly pure Milli-Q water (18 MΩ −1 cm −1 ) and reagent-grade chemicals, and the pH was adjusted using 1.0 M H 2 SO 4 and 1.0 M NaOH [35] . No agent for pH buffering was added to the electrolyte solution to avoid influences from the specific adsorption of multivalent anions. The prepared electrolyte solution was bubbled with Ar gas prior to measurements and temperature of the reactor was kept at 30 °C unless otherwise noted. For minimizing pH changes near the electrode surface, the j versus U curve was measured using a potential sweep from negative to positive without stirring. The amount of dissolved oxygen in the electrolyte solution was monitored simultaneously during the j versus U measurements using a needle-type oxygen microsensor (Microx TX3-trace, PreSens). A gas chromatograph equipped with a TCD detector (GC-8A, Shimadzu) was used to monitor the amount of oxygen in the head-space of electrochemical reactors. Pyridine and its derivatives were obtained from Wako, and isotopic reagents (D 2 O and D 2 SO 4 for pD adjustment) were purchased from Sigma-Aldrich. How to cite this article: Yamaguchi, A. et al. Regulating proton-coupled electron transfer for efficient water splitting by manganese oxides at neutral pH. Nat. Commun. 5:4256 doi: 10.1038/ncomms5256 (2014).